Carbon nanotube membranes with ultrahigh specific adsorption capacity for water desalination and purification Development of technologies for water desalination and purification is critical to meet the global challenges of insufficient water supply and inadequate sanitation, especially for point-of-use applications. Conventional desalination methods are energy and operationally intensive, whereas adsorption-based techniques are simple and easy to use for point-of-use water purification, yet their capacity to remove salts is limited. Here we report that plasma-modified ultralong carbon nanotubes exhibit ultrahigh specific adsorption capacity for salt (exceeding 400% by weight) that is two orders of magnitude higher than that found in the current state-of-the-art activated carbon-based water treatment systems. We exploit this adsorption capacity in ultralong carbon nanotube-based membranes that can remove salt, as well as organic and metal contaminants. These ultralong carbon nanotube-based membranes may lead to next-generation rechargeable, point-of-use potable water purification appliances with superior desalination, disinfection and filtration properties. Water treatment technologies, including water desalination and purification, are critical for addressing the issues of clean water shortage around the world [1] , [2] . Reverse osmosis (RO) [3] , [4] and thermal processes [5] are widely implemented in large-scale, industrialized desalination plants. However, large-scale plants consume a large amount of energy and involve high operating costs associated with infrastructure and skilled labour [6] , making them difficult to be implemented in developing countries and resource-limited areas. Smaller point-of-use (POU) potable water purification devices [7] , [8] , [9] , on the other hand, can avoid many of these obstacles and are increasingly recognized as one of the appropriate approaches to meet the needs of clean water and sanitation at the household and community levels. POU water purification systems often comprise materials that adsorb contaminants, the most common being activated carbons obtained by a variety of methods [10] . However, although activated carbons can effectively remove organic contaminants and heavy metals, their capacity to adsorb salts is limited, and there are currently only few techniques that can efficiently desalinate water at a small scale [3] . Development of materials with high salt adsorption capacity will enable the realization of simple POU systems for direct desalination and purification of brackish water. Recently, carbon nanotubes (CNTs) have emerged as promising nanomaterials in water purification and desalination devices, mainly owing to the advantageous features of fast water transport, large surface area, and ease of functionalization [11] , [12] , [13] , [14] , [15] , [16] , [17] , [18] , [19] , [20] . Water permeability through CNTs interiors could be at least three orders of magnitude higher than that predicted by the Hagen–Poiseuille equation [11] , [12] , [15] , thereby significantly reducing the energy consumption in water treatment. The most intriguing way of integrating CNTs into water purification and desalination devices is to use vertically aligned CNTs with functionalized open ends that allows water to pass through but rejects salt ions [15] , [16] , [17] , [18] , [19] , [20] . However, complex fabrication and the difficulty in obtaining CNTs with subnanometer diameters remain challenges. An alternative approach is to directly deposit CNTs onto a porous membrane and remove salt via capacitive electrostatic interactions [21] , [22] , [23] ; however, the salt adsorption capacity is limited [24] , [25] . Other methods, such as surface functionalization with carboxylic and alkoxysilane-based chemical groups, were also reported to enhance water flux and desalination efficiency of such CNT-based membranes, for example, as demonstrated in the case of membrane distillation [26] . Here we demonstrate that the plasma treatment of CNTs can result in ultrahigh capacity to adsorb salt. We construct an adsorptive membrane by depositing a thin layer of ultralong CNTs (UCNTs) onto a mixed cellulose ester (MCE) porous support. We show that by subsequently modifying the UCNTs with plasma, the membranes can effectively remove salt, organics and nanoparticles simultaneously from aqueous solutions. As salt is adsorbed rather than rejected, the required operation pressure is significantly less than that required for RO. The ultrahigh adsorption capacity is attributed to the plasma-mediated conversion of the outer layers of the UCNTs to an amorphous network. This work presents a new approach to realize carbon-based materials with ultrahigh specific adsorption capacity for salts. Fabrication and modification of UCNT membranes UCNTs were synthesized by a water-assisted chemical vapour deposition process [27] , [28] . Scanning electron microscopy (SEM) and transmission electron microscopy (TEM) images indicated that these UCNTs had a vertically aligned, closely packed structure with a height of 100–200 μm, a diameter of 5–20 nm and a typical wall number of 5–10 ( Fig. 1a and Supplementary Fig. S1 ). The UCNTs were then removed from the growth substrate and sonicated in an aqueous solution with a surfactant (SDS) to form the CNT ink. Membranes based on these UCNTs were fabricated by vacuum filtration technique [29] , where a conformal thin layer of UCNTs was deposited on the porous MCE support (pore size of ~220 nm; Fig. 1b ). The resultant UCNT-based membranes were mechanically robust and could be bent at an angle of 90° more than 20 times without damage or loss of structural integrity ( Fig. 1c ). 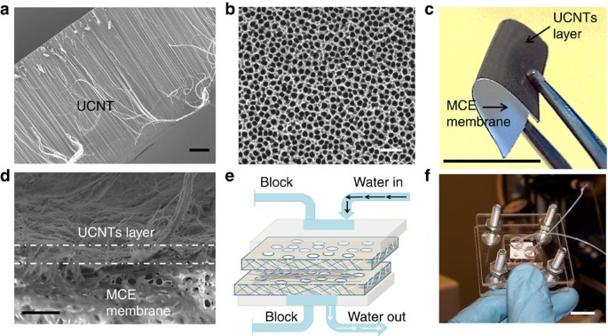Figure 1: UCNT-based membranes in micro-channel device. (a) Cross-sectional SEM image of the pristine UCNTs. Scale bar, 20 μm. (b) Top view: SEM image of the porous MCE support with an average pore size of 220 nm. Scale bar, 1 μm. (c) Photo of a UCNT–MCE membrane fabricated by vacuum filtration. Excellent flexibility of the membrane is demonstrated by the large-angle bending with no surface damage or structural degradation. Scale bar, 1 cm. (d) Cross-sectional SEM image of the pristine UCNT–MCE membrane. The thickness of the UCNT layer is ~0.5 μm. Scale bar, 1 μm. (e) Schematic diagram of the UCNT–MCE membrane integrated into a micro-cross channel device. Salt water flows through the channel with two identical membranes pressed face-to-face. (f) Photo of the actual micro-channel device. Scale bar, 1 cm. Figure 1d shows the cross-sectional images of the membrane, where a ~0.5-μm thick UCNT layer on the MCE support is clearly observed. The UCNT layer features a highly porous structure (~60% porosity; Supplementary Figs S2 and S3 ), which is desirable for effective water flow. Figure 1: UCNT-based membranes in micro-channel device. ( a ) Cross-sectional SEM image of the pristine UCNTs. Scale bar, 20 μm. ( b ) Top view: SEM image of the porous MCE support with an average pore size of 220 nm. Scale bar, 1 μm. ( c ) Photo of a UCNT–MCE membrane fabricated by vacuum filtration. Excellent flexibility of the membrane is demonstrated by the large-angle bending with no surface damage or structural degradation. Scale bar, 1 cm. ( d ) Cross-sectional SEM image of the pristine UCNT–MCE membrane. The thickness of the UCNT layer is ~0.5 μm. Scale bar, 1 μm. ( e ) Schematic diagram of the UCNT–MCE membrane integrated into a micro-cross channel device. Salt water flows through the channel with two identical membranes pressed face-to-face. ( f ) Photo of the actual micro-channel device. Scale bar, 1 cm. Full size image The membrane was then incorporated into a micro-channel device consisting of two identical membranes pressed together face-to-face to form the filtration section ( Fig. 1e and f ). Before device assembly, we modified the UCNTs via acid or plasma to investigate the correlation between the surface functionalities and the desalination efficiency (see Methods ). 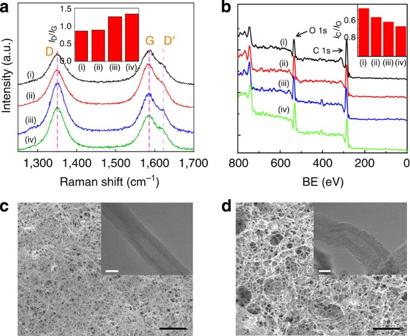Figure 2: Surface properties of UCNT–MCE membranes. (a) Raman and (b) XPS spectra of four different UCNT membranes used in the experiments: (i) pristine, (ii) acid modified, (iii) 5-min plasma-modified and (iv) 10-min plasma-modified membranes. Raman D, G and D’ peaks are labelled inaand XPS C 1 s and O 1 s peaks are labelled inb. Inset ofaplots theD/Gpeak intensity ratio (ID/IG) of the four samples and inset ofbplots the C/O peak intensity ratio (IC/IO). Top view: SEM image of (c) pristine and (d) plasma-modified (with 10-min plasma treatment) UCNT membranes. The insets ofcanddare high-resolution TEM images of a typical single UCNT before and after plasma (10-min treatment), respectively. The lattice spacing between the two atomic layers is measured to be 0.34 nm. The typical wall numbers of the UCNT are about 10 to 12. Scale bars, 2 μm. Inset scale bars, 5 nm. Figure 2a shows the resonant micro-Raman spectra of all the UCNT–MCE membranes used in the experiments. In these spectra, the G peak at 1,584 cm −1 can be assigned to the phonon mode E 2g in CNTs, which involves the out-of-phase intralayer displacements; the D (at 1,350 cm −1 ) and D’ (at 1,622 cm −1 ) peaks correspond to the disorder-induced phonon modes arising from the finite size of the crystals and defects, respectively [30] . The positions of these peaks remained essentially unchanged for pristine and acid/plasma-modified UCNT–MCE membranes. However, the relative intensities of the D and G peaks (that is, I D / I G ratio), which is generally used to determine the impurity and structural quality of CNTs [31] , increased from 0.8 for the pristine membrane to 1.26 for the plasma-modified one (inset of Fig. 2a ). This indicated that more defective structures were induced on the UCNTs by the plasma modification [32] . Figure 2: Surface properties of UCNT–MCE membranes. ( a ) Raman and ( b ) XPS spectra of four different UCNT membranes used in the experiments: (i) pristine, (ii) acid modified, (iii) 5-min plasma-modified and (iv) 10-min plasma-modified membranes. Raman D, G and D’ peaks are labelled in a and XPS C 1 s and O 1 s peaks are labelled in b . Inset of a plots the D / G peak intensity ratio ( I D / I G ) of the four samples and inset of b plots the C/O peak intensity ratio ( I C /I O ). Top view: SEM image of ( c ) pristine and ( d ) plasma-modified (with 10-min plasma treatment) UCNT membranes. The insets of c and d are high-resolution TEM images of a typical single UCNT before and after plasma (10-min treatment), respectively. The lattice spacing between the two atomic layers is measured to be 0.34 nm. The typical wall numbers of the UCNT are about 10 to 12. Scale bars, 2 μm. Inset scale bars, 5 nm. Full size image The above Raman analysis was further verified by X-ray photoelectron spectroscopy (XPS). As shown in Fig. 2b , the intensity ratio between C1s and O1s peaks of the pristine UCNT–MCE membrane (that is, I C /I O ratio) decreased after plasma modification. The corresponding C1s narrow scans revealed that more oxygen-containing bonds, such as the hydroxylic (−OH) and carboxylic (–COOH) surface groups, were formed in the plasma-modified samples ( Supplementary Fig. S4 ). These results unambiguously indicated that the plasma had introduced surface functional groups and altered the UCNT structure, which in turn had an important role in the adsorption-based water desalination and filtration. Characterization of the morphology and structure of the UCNT layers before and after plasma modification by SEM and TEM revealed that the pristine UCNTs were synthesized with a high quality ( Fig. 2c ). Few amorphous carbon structures were detected and highly ordered graphitic structures were found in the corresponding TEM images. On the other hand, the UCNT–MCE membranes after 5- or 10-min plasma treatment exhibited severe structural damage on the outer layers where the graphitic walls were no longer evident ( Fig. 2d ), which is consistent with the above Raman and XPS results. The structure of UCNTs was not completely destroyed in the plasma surface modification process; instead, the outer layers of UCNTs were modified ( Supplementary Fig. S3 ). Desalination using UCNT membranes The desalination performance of the pressure-driven micro-channel device was evaluated by measuring the conductivity change of salt water after flowing through the device with a single inlet and outlet ( Fig. 1e ). The entire system, including the upstream and downstream volumes, was initially filled with NaCl solution (3,500 p.p.m. or 0.06 M). Prefilling with the saline solution was employed to avoid bubble entrapment and to exclude any fresh water from the system, so that any change in conductivity could be directly related to the removal of salt by the UCNTs. The solution was then pumped through the device and the real-time salt concentration of the output stream was monitored. 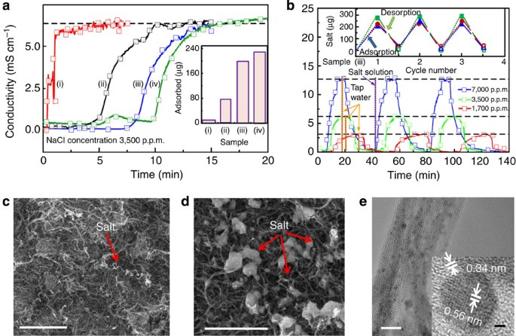Figure 3: Salt removal by UCNT–MCE membranes. (a) Conductivity curves for the passage of 3,500 p.p.m. NaCl solutions through the micro-channel device using four membranes: (i) pristine, (ii) acid-modified, (iii) 5-min plasma-modified and (iv) 10-min plasma-modified membranes. Inset inashows the mass of salt removed by each membrane. (b) Plot of the conductivity of three adsorption–desorption cycles using sampleivat NaCl concentrations of 7,000, 3,500 and 1,700 p.p.m. Inset inbshows the mass of salt removed in each cycle. (c) SEM image of sampleiafter the adsorption reaches saturation. Scale bar, 1 μm. (d) SEM image of sampleivafter the adsorption reaches saturation. More NaCl nanocrystals are observed on sampleiv. Scale bar, 1 μm. (e) TEM image of scattered NaCl nanocrystals in sampleiv. Scale bar, 20 nm. Inset ineshows the crystal lattice of NaCl NPs embedded in the UCNT networks. Scale bar, 1 nm. Figure 3a plots the conductivity curves of salt water after passing through the four different membranes ( Supplementary Table S1 ). The conductivity of salt water flowing through the pristine UCNT–MCE membrane (that is, sample i ) first decreased and then rapidly increased to reach a stabilized value of the initial NaCl solution within a short period of time (<1 min). In contrast, the conductivity remained at a significantly low level for the acid-modified UCNT–MCE membrane (that is, sample ii ). Only after 5 min, the conductivity started to increase and finally reached the feed concentration value. For the plasma-modified membranes (that is, samples iii and iv ), the conductivity did not start to rise until 7.5–10 min, and the stabilized value was reached only after 13–15 min. Figure 3: Salt removal by UCNT–MCE membranes. ( a ) Conductivity curves for the passage of 3,500 p.p.m. NaCl solutions through the micro-channel device using four membranes: (i) pristine, (ii) acid-modified, (iii) 5-min plasma-modified and (iv) 10-min plasma-modified membranes. Inset in a shows the mass of salt removed by each membrane. ( b ) Plot of the conductivity of three adsorption–desorption cycles using sample iv at NaCl concentrations of 7,000, 3,500 and 1,700 p.p.m. Inset in b shows the mass of salt removed in each cycle. ( c ) SEM image of sample i after the adsorption reaches saturation. Scale bar, 1 μm. ( d ) SEM image of sample iv after the adsorption reaches saturation. More NaCl nanocrystals are observed on sample iv . Scale bar, 1 μm. ( e ) TEM image of scattered NaCl nanocrystals in sample iv . Scale bar, 20 nm. Inset in e shows the crystal lattice of NaCl NPs embedded in the UCNT networks. Scale bar, 1 nm. Full size image The mass m of salt removed by each membrane can be calculated based on the conductivity curves and the flow rate [33] where C 0 is the initial salt concentration, C t is the real-time salt concentration determined from the electrical measurement, and V is the volume of the solution flowed. We found that ~8 μg (~18% w/w) of salt was removed by the pristine UCNT–MCE membrane (sample i ; inset of Fig. 3a ). This amount of salt removal significantly increased to ~60 μg for the acid-modified membrane (sample ii ; inset of Fig. 3a ). The maximum salt removal was observed on the two plasma-modified samples iii and iv (inset of Fig. 3a ) with ~180 and ~225 μg of salt removal, respectively. Considering that the total mass of UCNTs that contributed to the water desalination process was only about 45 μg, the adsorption capacity of the plasma-modified UCNTs (defined as the total removed salt divided by the total weight of UCNTs) is therefore at least 400% w/w (that is, 4 g g −1 or 4,000 mg g −1 ). The amount of salt that can be removed by the activated carbons reported in the literature is around 2–20 mg g −1 (or 0.2–2% w/w) [10] . Therefore, the adsorption capacity of plasma-modified UCNTs is about two orders of magnitude higher than that of activated carbons. The amount of salt removal is also notably higher than the adsorption capacity of the state-of-the-art porous carbon materials (~15 mg g −1 or 1.5% w/w) used in the capacitive deionization [34] . Validation of ultrahigh adsorption capacity To further elucidate the ultrahigh specific adsorption capability of sample iv , the above experiment was repeated with the NaCl solution at varied concentrations of 7,000, 3,500 and 1,700 p.p.m. Interestingly, the plasma-modified membrane iv could achieve a 100% recovery of its salt-removal capability simply by rinsing with tap water (conductivity ~500–600 μS cm −1 , hardness ~0.0513, kg m −3 and chlorine level ~3 p.p.m.) following a maximum adsorption, that is, a stabilized conductivity in the curves ( Fig. 3b ). One can see that at a higher NaCl concentration, the adsorption reached its maximum value faster than that at a lower concentration. The total amount of salt removed, however, was relatively constant regardless of the salt concentration (inset of Fig. 3b ). This independence between the salt removal and the concentration (that is, ionic strength) of the salt solution further confirmed the proposed adsorptive mechanism. If the salt removal was dominated by electrostatic repulsion or electrokinetic effects, the desalination capacity would be sensitive to the ionic strength and the Debye screening length [17] , but a constant amount of salt would be removed if the UCNTs had a high affinity for salt adsorption. The adsorbed salt on the surface of different UCNT membranes was further visualized by SEM. As shown in Fig. 3c,d , only a few NaCl crystals were observed on the surface of the pristine sample i , whereas a significantly higher density of NaCl crystals was found on the plasma-modified sample iv . Small NaCl crystals presumably on the defective sites and possibly penetrating within the UCNTs, were also observed in the high-resolution TEM image ( Fig. 3e and Supplementary Fig. S5 ); the crystal lattice could be clearly identified (inset of Fig. 3e ). These observations further suggest that the UCNT-based membranes did not operate as a semipermeable medium to filter the salt (that is, the mechanism of RO membranes); instead, they utilized the ultrahigh adsorption capacity to remove salt from the solution. Given that the density of the UCNT layer is in the range of 0.4 to 0.8 g cm −3 and that of the UCNTs is 1.4 g cm −3 , ~60% of its volume is empty space. As the density of NaCl crystals is 2.17 g cm −3 , the volume occupation of salt adsorbed is estimated to be ~70% of that of the UCNT layer, which agrees well with the microscopic observations ( Fig. 3d and Supplementary Fig. S5 ). We attribute this high adsorption capability of samples iii and iv to the numerous defective sites created by the plasma treatment. The high-resolution TEM images suggest that the plasma treatment significantly damaged the UCNTs, making the outer layers amorphous and possibly porous ( Fig. 2d and Supplementary Fig. S5 ). Strong acid or plasma is known to partially damage the graphitic structure of CNTs and create dangling bonds, which then react with the ambient gases to form various functional/charged groups, particularly the oxygen-containing groups, such as –COOH and –OH [17] . The above Raman and XPS analyses confirmed the presence of these functional groups on the acid-/plasma-modified UCNTs ( Fig. 2 ). In combination with a high surface area, these functional groups could greatly enhance surface hydrophilicity and ion-binding properties of the modified UCNTs. In addition, with a small (~10 nm) UCNT diameter, their modified outer layers are easily accessible to the solution. Consequently, a high salt adsorption capability was achieved with the modified UCNTs when salt water flowed through the porous structure [35] , [36] . It is worth mentioning that samples ii – iv could completely remove salt below the detection threshold of 10 –7 M from the solution in the first round of the filtration process (shown in Fig. 3a in the first 5 min), whereas little salt was removed for the pristine UCNT–MCE membranes. The nearly complete removal of salt implied an excellent mass transfer from the solution to the UCNTs. Assuming a maximum pore size of 200 nm, a UCNT layer thickness of 500 nm and a flow velocity of 5 × 10 –5 m s −1 , the Péclet number ( P e =ν L / D , where ν is the flow velocity, L is the characteristic length and D is the diffusion coefficient of sodium ions), which defines the ratio of convective to diffusive mass transfer, is estimated to be 2.5 × 10 –4 . As P e <<1, it is expected that diffusion will be sufficient to ensure salt adsorption as the solution flows through the UCNT layer. Removal of organics and metal nanoparticles An efficient water membrane should also be capable of effectively removing organic or inorganic contaminants linking to waterborne diseases, including biomolecules, microorganisms and heavy metals. To verify such capability of the current UCNT–MCE membranes, we used sample iv as an example to filter dextran molecules ( M w =70,000) labelled with rhodamine. The aqueous solution of these fluorescent rhodamine-dextran (RD) conjugates was filtered through the same micro-channel device and the concentration of RD in the filtered water was determined by ultraviolet–visible spectrophotometry. To examine the effect of charges on RD molecules (pK a ~6.4) [18] , the solution’s pH value was also adjusted to 4 or 7. 100 μl aliquots were collected during the filtration process. The absorption spectra of water with RD at pH 7 and 4 first decreased in intensity, and then increased gradually as the filtration progressed ( Fig. 4a,b ). The absorption peak intensity (that is, ~514 nm) of filtered solution decreased sharply in the first few aliquots; it then recovered to the value of fresh RD solution at longer times ( Fig. 4c ). Fluorescence microscopic analysis of the membranes revealed that the UCNTs were fully covered with RD molecules after filtration (inset in Fig. 4c ). Arguably, the adsorption capability was stabilized in a slower manner in the RD solution at pH 4 ( Fig. 4c ), suggesting that the charge on the molecules may also have a role in the interactions with the UCNTs. 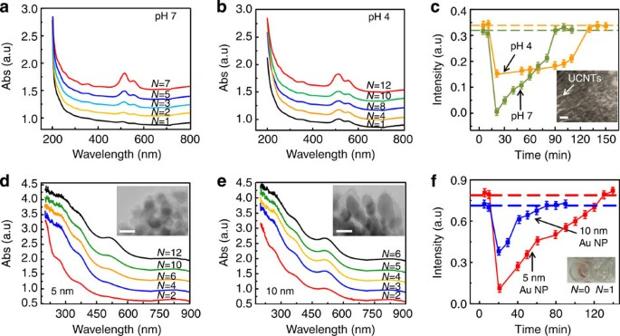Figure 4: Removal of RD and gold NPs by UCNT–MCE membrane. aandbshow the adsorption spectra of 100-μl aliquots collected sequentially during filtration of the RD solutions at pH 7 and 4, respectively. (c) Adsorption intensity of filtered RD solutions at 514 nm. Data represent mean±s.e. of three independent experiments. Inset incis the microscopic florescence image of the membrane after 50-min filtration. Scale bar, 500 μm.dandeare the adsorption spectra of the solutions containing gold NPs with diameters of 5 and 10 nm, respectively. Insets indandeare the TEM images of gold NPs adsorbed on the corresponding membranes after 50-min filtration. Scale bars, 5 nm and 10 nm, respectively. (f) Adsorption intensity of filtered solutions of gold NPs at 521 nm. Data represent mean±s.d. of three independent experiments. Inset infshows the photos of water dispersed with 5-nm gold NPs before and after filtration (the first aliquot). The colour changed from red to transparent, indicating that almost all the NPs were removed by the UCNT membrane. N denotes the aliquot number. Figure 4: Removal of RD and gold NPs by UCNT–MCE membrane. a and b show the adsorption spectra of 100-μl aliquots collected sequentially during filtration of the RD solutions at pH 7 and 4, respectively. ( c ) Adsorption intensity of filtered RD solutions at 514 nm. Data represent mean±s.e. of three independent experiments. Inset in c is the microscopic florescence image of the membrane after 50-min filtration. Scale bar, 500 μm. d and e are the adsorption spectra of the solutions containing gold NPs with diameters of 5 and 10 nm, respectively. Insets in d and e are the TEM images of gold NPs adsorbed on the corresponding membranes after 50-min filtration. Scale bars, 5 nm and 10 nm, respectively. ( f ) Adsorption intensity of filtered solutions of gold NPs at 521 nm. Data represent mean±s.d. of three independent experiments. Inset in f shows the photos of water dispersed with 5-nm gold NPs before and after filtration (the first aliquot). The colour changed from red to transparent, indicating that almost all the NPs were removed by the UCNT membrane. N denotes the aliquot number. Full size image The plasma modified UCNT–MCE membrane is also capable of removing heavy metal nanoparticles (NPs). To demonstrate this, sample iv was again used to filter water dispersed with gold NPs. Optical absorbance of the filtered water with gold NPs with average diameters of 5 and 10 nm, respectively, show effective removal of the gold NPs ( Fig. 4d,e ). Gold NPs embedded in the UCNT networks were also observed in TEM images (insets in Fig. 4d,e ). Figure 4f plots the peak intensity (at 521 nm) of water dispersed with gold NPs as the filtration progressed. The plots show that gold NPs with a smaller size can be removed more effectively than their larger counterparts. This result is contradictory to the size-selective mechanism commonly observed in many porous membranes, where the passage of small-sized NPs is preferred. However, it is consistent with the proposed adsorptive mechanism. In the case of small-sized gold NPs, the interactions between the surface defective sites on the UCNTs and the NPs are substantially stronger [32] , leading to higher retention efficiency. In contrast, the relatively weaker interactions on larger gold NPs were less effective in retaining them [37] . Static salt adsorption by CNT-based membranes To further verify the high adsorption capacity of plasma-modified UCNT–MCE membranes, we studied the adsorption behaviour of the four types of membranes ( i – iv , 1 cm 2 area) in static salt water (0.02 M or 1,167 p.p.m. NaCl). 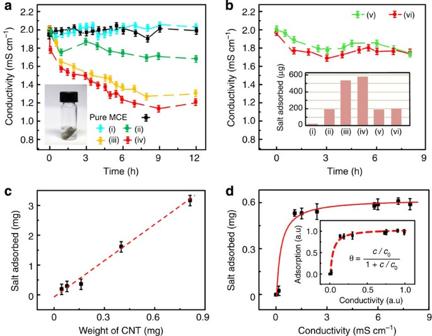Figure 5: Adsorption tests in static salt water. (a) The plots of conductivity changes in static salt water when membranes are immersed in 1 ml of 0.02 M salt water. Membranes include: pure MCE, (i) pristine UCNT–MCE, (ii) acid-modified UCNT–MCE, (iii) 5-min plasma-modified and (iv) 10-min plasma-modified UCNT–MCE. Inset inashows a photo of the membrane immersed in the salt solution. (b) Conductivity changes in static salt water using short MWCNT-based membranes: (v) pristine MWCNT–MCE and (vi) 10-min plasma-modified MWCNT–MCE. Inset inbplots the amount of salt adsorbed for all membranes inaandb. (c) Salt adsorbed for 10 min by plasma-modified UCNT–MCE with different UCNT mass in 0.02 M salt water and (d) for 160 μg of UCNT–MCE in salt water with different conductivities. Inset indshows the Langmuir isotherm equation fitting plot of the experiment results, where theθis the mass of salt adsorbed normalized by the total salt adsorption capacity,cis the normalized conductivity of the salt water at equilibrium andc0is the Langmuir adsorption constant. Data represent mean±s.d. of three independent experiments. Figure 5a shows the conductivity changes of the salt water as a function of the immersion time. By converting the conductivity changes to the mass of salt removed, the adsorption capacity of sample iv was found to be 590 μg with 160 μg of UCNTs immersed ( Fig. 5b ), which was the highest value among the four membranes. This result is in a good agreement with the 400% w/w specific adsorption observed in the micro-channel filtration experiments. In comparison, the pristine UCNT-based membrane (sample i ) and the pure MCE membrane showed adsorption of <20 μg (inset of Fig. 5b ). These results therefore confirmed that the plasma treatment is essential for an enhanced salt adsorption of the UCNT-based membranes. Figure 5: Adsorption tests in static salt water. ( a ) The plots of conductivity changes in static salt water when membranes are immersed in 1 ml of 0.02 M salt water. Membranes include: pure MCE, (i) pristine UCNT–MCE, (ii) acid-modified UCNT–MCE, (iii) 5-min plasma-modified and (iv) 10-min plasma-modified UCNT–MCE. Inset in a shows a photo of the membrane immersed in the salt solution. ( b ) Conductivity changes in static salt water using short MWCNT-based membranes: (v) pristine MWCNT–MCE and (vi) 10-min plasma-modified MWCNT–MCE. Inset in b plots the amount of salt adsorbed for all membranes in a and b . ( c ) Salt adsorbed for 10 min by plasma-modified UCNT–MCE with different UCNT mass in 0.02 M salt water and ( d ) for 160 μg of UCNT–MCE in salt water with different conductivities. Inset in d shows the Langmuir isotherm equation fitting plot of the experiment results, where the θ is the mass of salt adsorbed normalized by the total salt adsorption capacity, c is the normalized conductivity of the salt water at equilibrium and c 0 is the Langmuir adsorption constant. Data represent mean±s.d. of three independent experiments. Full size image To demonstrate the critical role that UCNTs had in the adsorption, commercial multi-walled CNTs (MWCNTs) were also employed to construct the membranes using the same procedures. These MWCNTs had a comparable diameter of 5–20 nm but a substantially shorter length of 10 μm ( Supplementary Fig. S6 ). Figure 5b shows the adsorption kinetic tests in static salt water, where samples v and vi represent the pristine and plasma-modified short CNT-based membranes, respectively. It is found that both membranes exhibited a similar adsorption behaviour with the same amount of salt removal of ~200 μg (inset of Fig. 5b ). This adsorption capacity was higher than that of the pristine UCNT membranes, but was significantly lower than that of the plasma-modified UCNT samples. Microscopic analyses indicated that in contrast to the UCNT layer, a much sparse structure of the top MWCNT layer was formed on the porous MCE support ( Supplementary Fig. S8 ). This is possibly because of the short length of MWCNTs, which provided insufficient van der Waals’ forces to bundle them firmly [38] and were too short to form a layer similar to that of the much longer UCNTs. Furthermore, XPS spectra revealed that plasma was not so effective in introducing defective sites on these MWCNTs ( Supplementary Figs S6 and S7 ). The sparse structure and the less defective sites could therefore be responsible for the moderate adsorption capacity observed on these short CNT-based membranes. To further study the adsorption characteristics of the UCNTs, we synthesized 10 min plasma-treated UCNT–MCE membrane with different UCNT masses and immersed the samples in static salt water (0.02 M or 1,167 p.p.m. NaCl). As shown in Fig. 5c , the specific adsorption results are in a close agreement with 400% w/w adsorption capacity. Next, we tested the adsorption capacity of 160 μg UCNT–MCE membrane in salt water at different concentrations. The removed salt as a function of the final solution concentration fitted well to the Langmuir adsorption isotherm ( Fig. 5d ): where the θ is the mass of salt adsorbed normalized by the total salt adsorption capacity, c is the salt concentration and c 0 is the Langmuir adsorption constant. This curve shows that the 10 min plasma-treated UCNT–MCE membrane has a corresponding c 0 of ~250 p.p.m. (4.3 mM), that is, half the adsorption capacity of the UCNTs is attained at 250 p.p.m. Knowing this value, we can estimate the interfacial energy change involved in salt adsorption. For precipitation of a thin layer of salt on a surface, the work of precipitation W is given by [39] where n is the number of salt molecules precipitated, S is the ratio of the actual activity of the salt to that of salt at saturation, Δ γ is the net change in interfacial energy per unit area, v 0 is the molecular volume and t is the thickness of the precipitated crystal ( nv 0 / t is the area). Assuming that the surface on which adsorption occurs is nearly covered when the salt concentration is 10 mM, setting the work of precipitation to zero at that concentration (that is, assuming equilibrium) yields Δ γ ~0.025 N m −1 for t =0.2 nm and Δ γ ~0.125 N m −1 for t =1 nm. This order of magnitude of surface energy is within the range of typical interfacial energies (for example, surface energy of NaCl crystals is ~0.4 N m −1 ) (ref. 40 ), suggesting that the observed Langmuir adsorption may be explained by the high surface energy of the plasma-treated UCNTs. This observed salt adsorption may be similar to capillary condensation, where crystals of salt can form on surfaces or in confined spaces below saturation concentrations due to the high surface energy of the interfaces [41] . The exact mechanism of the salt adsorption, namely the structure of the adsorbed salt and to what extent it penetrates into the layers of the UCNTs to result in the remarkable adsorption capacity, presents an intriguing question that will require further investigations. The main criteria in the development of portable POU water desalination systems include the cost, efficiency, usability and the ability to simultaneously desalinate and purify contaminated water. The feasibility of using such systems in remote areas without a continuous power supply is also practically important. To this end, we have demonstrated the high performance of plasma-modified UCNT-based porous membranes in the removal of salt, organic molecules and metal NPs from low to medium salinity solutions. As compared with the currently available water desalination techniques, the advantages of using the UCNT-based membranes with ultrahigh adsorption capability are obvious: RO requires high pressure, and neither electrodialysis nor capacitive deionization is suited for the removal of organic chemicals unless an additional barrier is used. Furthermore, RO systems cannot be carried easily on person, so that their mobility is limited. Although POU RO desalination systems have recently become available, issues associated with the common RO membranes remain, that is, low water flux, high energy and operational cost, and the inability to remove organics and some heavy metal contaminants [4] , [9] . In contrast, the driving force for desalination of UCNT-based membranes is the free energy of adsorption and only a small pressure drop is required to provide sufficient water flux to ensure fast convection of salt to the UCNTs. The UCNTs can simultaneously desalinate water and remove organic/inorganic contaminants, and the porous MCE membrane can filter out microbes. We anticipate that devices made from the UCNT membranes may operate as a rechargeable cartridge, similar to a battery. The devices could be carried on person to provide clean water and could be recharged at a station where fresh water is available. For example, about 100 L of brackish water (10,000 p.p.m.) could be purified by 250 g of the UCNTs. Results of ultrahigh adsorption capability of UCNT-based membranes were mainly obtained from low salinity water. Some practical issues may arise for desalination of real seawater with complex ionic makeup. In certain zeolite exchange-based desalination systems, the divalent ions (for example, Mg 2+ , Ca 2+ ) with higher charge densities might block sites for the monovalent ions when the systems allow them to enter the porous structure equally [42] . Further investigations are thus needed to elucidate whether the UCNT-based membranes are suited for other applications besides those discussed above. In conclusion, we have demonstrated that plasma-treated UCNTs display a remarkably high capacity for adsorption of salt, which opens the possibility of desalination via salt adsorption. This adsorption capacity was easily recovered by rinsing with tap water. Furthermore, the UCNTs could also adsorb organics and NPs. Devices made using these membranes may be useful for POU purification of brackish water, operating like rechargeable cartridges. Although the exact mechanism of salt adsorption is not fully understood, further studies may provide insight into design of materials with ultrahigh adsorption capacity for a variety of applications. Synthesis of UCNTs Vertically aligned UCNTs were synthesized by water-assisted chemical vapour deposition process as reported previously [27] , [28] . Briefly, a 0.5-nm thick Fe catalyst film was deposited on n -type Si substrate coated with Al 2 O 3 and SiO 2 interlayers with a thickness of 10 and 100 nm, respectively. The catalyst was then annealed to 750 °C under an Ar/H 2 (900/600 sccm) mixture at atmospheric pressure. The growth of CNTs was started by introducing C 2 H 4 at a flow rate of 600 sccm and a trace amount of water. After typically 10 min, the growth was terminated and the furnace was cooled down to room temperature. UCNTs with an average of 5–10 walls and a height of 100–200 μm were obtained ( Supplementary Fig. S1 ). Fabrication and modification of UCNT-based membranes To fabricate the membranes, the vertically aligned UCNTs were removed from the silicon substrate and dispersed in 1 wt% SDS solution. The solution was sonicated for 30 min using a tip-sonicator (Sonics VCX1F30) to yield a stable and uniformly dispersed UCNT ink. The UCNT ink was then deposited onto the commercially available MCE porous membranes (Millipore GSWP04700) with a size ~10 cm 2 by vacuum filtration [29] . The residual surfactant in the UCNT–MCE membrane was removed by filtering with copious tap water. After drying completely in a vacuum oven, the UCNT–MCE membrane was weighed by a balance (sensitivity ~0.01 mg; Mettier H20T) and the density of UCNTs on the membrane was estimated (0.4–0.8 g cm −3 ). The porosity was therefore ~60% by assuming that the density of bulk CNTs is 1.4 g cm −3 . Further microscopic images indicated that the homogeneous CNT film conformed well to the MCE membrane with a thickness of ~0.5 μm ( Supplementary Fig. S8 ). Both acid and plasma modification were conducted to functionalize the UCNT-based membranes. For acid modification, the membranes were immersed into 5 N HNO 3 , refluxed for 2 h and then washed with deionized water. For plasma modification, the membranes were placed in a plasma chamber with a ‘remote’ inductively coupled plasma configuration ( Supplementary Fig. S3 ). The plasma was generated by a radio frequency power operated at frequency of 13.56 MHz and power of 600 W, with 40 sccm Ar gas at a pressure of 2 Pa. The distance between the centre of the plasma and the UCNT–MCE membranes was ~40 cm. The modification time lasted for 5 and 10 min, respectively. Micro-channel and static water tests To test the desalination performance of membranes, the micro-channel device as shown in Fig. 1f was used. First, the UCNT–MCE membranes were cut into small pieces with an area of 1 × 1 cm 2 . Two identical pieces were then pressed face-to-face in the micro-channel device. The entire micro-channel device, connecting tubing and a precalibrated microfluidic conductivity measurement device comprising the fixed channel geometry (volume ~100 μl) and the embedded Ag/AgCl electrodes were first filled with the NaCl solution. The microfluidic device was then opened and the UCNT membrane was loaded into the device. The NaCl solution was then pumped through the device by a syringe pump (Harvard Apparatus, PHD 2200) at a flow rate of 10 μl min −1 . After allowing for 140 μl of the volume to flow (corresponding to the dead volume in the system), the conductivity of the outlet was monitored by measuring the conductance of the microfluidic device. No membrane clogging was found throughout the desalination operations. For the purification of RD molecules, 2.5 mg ml −1 solution was prepared in deionized water and the pH of the solution was adjusted to 7 (neutral) or 4 (anionic), respectively. The entire system was first filled with the RD solution, and a fresh UCNT membrane was loaded into the device. The RD solution was then flowed through the membrane at a flow rate of 10 μl min −1 . Every 10 min, 100-μl aliquots were collected in a vial and were analysed by a ultraviolet–visible spectrophotometer. For the filtration of gold NPs, solutions of gold NPs with a diameter of 5 nm (5.47 × 10 13 NPs per ml) and a diameter of 10 nm (5.98 × 10 12 NPs per ml) were used in the micro-channel device, and the same procedure as that for RD was followed. Finally, to measure the adsorption capacity of the membranes in static salt water, two identical samples of each membrane (1 × 1 cm 2 ) were immersed into 1 ml of salt water at a concentration of 0.02 M (inset of Fig. 5a ). The 10-min plasma-treated UCNT–MCE membrane with different UCNT masses were also synthesized and immersed in static salt water (0.02 M NaCl). The corresponding conductivities were then monitored every 30 min by an electrometer. Characterization techniques Field-emission SEM was performed using a Zeiss Auriga microscope operated at 1 keV electron beam energy with an InLens secondary electron detector. Vertical alignment of UCNTs was viewed by scratching the surface with tweezers. TEM was performed using a Philips CM120 with the electron beam energy of 120 keV (for low resolution) or a JEOL 2010 with the electron beam energy of 200 keV (for high resolution). The TEM samples were prepared by dispersing the grown nanotubes into ethanol and then dispersed onto the holey carbon-coated copper grids and dried in air. Raman spectroscopy was performed using a Renishaw inVia spectrometer with laser excitations at 514 nm and a probing spot size of ~1 μm 2 . XPS (Specs SAGE 150) used the Mg Kα excitation at 1,253.6 eV. Ultraviolet–visible spectra of the solution were carried out on a Lambda 35 spectrophotometer. How to cite this article: Yang, H. Y. et al . Carbon nanotube membranes with ultrahigh specific adsorption capacity for water desalination and purification. Nat. Commun. 4:2220 doi: 10.1038/ncomms3220 (2013).